Genome-wide identification of microRNA expression quantitative trait loci Identification of microRNA expression quantitative trait loci (miR-eQTL) can yield insights into regulatory mechanisms of microRNA transcription, and can help elucidate the role of microRNA as mediators of complex traits. Here we present a miR-eQTL mapping study of whole blood from 5,239 individuals, and identify 5,269 cis- miR-eQTLs for 76 mature microRNAs. Forty-nine per cent of cis- miR-eQTLs are located 300–500 kb upstream of their associated intergenic microRNAs, suggesting that distal regulatory elements may affect the interindividual variability in microRNA expression levels. We find that cis- miR-eQTLs are highly enriched for cis- mRNA-eQTLs and regulatory single nucleotide polymorphisms. Among 243 cis- miR-eQTLs that were reported to be associated with complex traits in prior genome-wide association studies, many cis- miR-eQTLs miRNAs display differential expression in relation to the corresponding trait (for example, rs7115089, miR-125b-5p and high-density lipoprotein cholesterol). Our study provides a roadmap for understanding the genetic basis of miRNA expression, and sheds light on miRNA involvement in a variety of complex traits. MicroRNAs (miRNAs), a class of small noncoding RNAs, serve as key post-transcriptional regulators of gene expression and mRNA translation [1] , [2] . miRNAs are increasingly recognized as mediators in a variety of biological processes including cardiovascular development and disorders [3] , [4] . Highly specific miRNA expression patterns have been reported in association with heart failure [5] , [6] , myocardial infarction [7] and cancer [8] . However, the influence of genetic variation on miRNA expression and function still remains unclear. Recently, many genome-wide expression quantitative trait locus (eQTL) mapping studies have revealed common genetic loci associated with mRNA expression levels of many genes [9] , [10] , [11] , [12] . These eQTL analyses have demonstrated that transcript levels of many mRNAs behave as heritable quantitative traits. In contrast to more extensive investigations of mRNA eQTLs in multiple tissues [13] such as blood [9] , brain [10] , fat [11] and liver [12] , there are relatively few studies of miRNA eQTLs (miR-eQTLs) and those that have been published to date are based on modest sample sizes ( n <200) [14] , [15] , [16] , [17] , [18] . These studies have identified relatively few cis -miR-eQTLs; uncertainty persists regarding the number of miR-eQTLs in humans and their relations to regulatory elements in the human genome. We conduct a genome-wide miR-eQTL study by utilizing genome-wide genotypes and miRNA expression profiling of whole blood derived RNA from 5,239 Framingham Heart Study (FHS) participants. We analyze the associations of ~10 million 1000 Genomes Project [19] imputed single nucleotide polymorphisms (SNPs) (at minor allele frequency (MAF) >0.01 and imputation quality ratio >0.1) with whole blood-derived miRNA expression levels of 280 mature miRNAs expressed in >200 individuals, representing 11% of all discovered human miRNAs to date (2,576 mature miRNAs have been reported in miRbase v20: www.mirbase.org ). We calculate both cis- and trans- miR-eQTLs genome wide, and identify cis -miR-eQTLs with concordant effects in two pedigree independent study groups. By cross-linking cis -miR-eQTLs SNPs with regulatory SNPs annotated by the ENCODE project [20] and with complex trait-associated SNPs identified in prior genome-wide association studies (GWAS) [21] , [22] , and by linking cis -miR-eQTL miRNAs with differentially expressed miRNAs for complex traits, we sought to dissect the genetic regulation of miRNA expression and explore the extent to which cis -miR-eQTLs may affect interindividual phenotype variability. Heritability of global miRNA expression in peripheral blood The demographic and clinical characteristics of the 5,239 FHS participants included in our analysis are shown in Supplementary Data 1 . The pedigree structure formed by these participants is shown in Supplementary Data 2 . We detected 280 mature miRNAs that were expressed in >200 participants (these miRNAs were used for identification of miR-eQTLs and unless specifically stated, miRNAs mentioned in the results and discussion refers to mature miRNAs), of these 247 miRNAs were expressed in >1,000 participants ( Supplementary Fig. 1 ). The distribution of narrow-sense heritability of miRNA expression for the 247 miRNAs expressed in >1,000 participants is shown in Supplementary Fig. 2 , with an average heritability estimate ( ) of 0.11; 133 miRNAs (54%) had and 9 miRNAs (miR-100-5p, miR-668, miR-133a, miR-127-3p, miR-409-3p, miR-20a-3p, miR-941, miR-191-3p and miR-1303) had (details in Supplementary Data 3 ). Cell type effects and reproducibility of miR-eQTLs To evaluate whether blood cell type proportions significantly influence miR-eQTLs, we compared miR-eQTLs identified in 2,138 FHS third generation cohort participants (in whom differential cell counts and proportion data were available) with and without adjustment for measured blood cell counts and cell type proportions (see Methods). Cell types did not appreciably influence miR-eQTLs ( Supplementary Fig. 3 ), however, we cannot exclude the possibility of small cell type effects. In the subsequent sections, we focus on miR-eQTLs from analyses that were unadjusted for cell counts of 5,239 individuals ( Supplementary Data 4 ). The miR-eQTLs from the model that adjusted for imputed cell counts in the larger set of 5,024 participants are provided in Supplementary Data 5 . To evaluate the reproducibility of detected miR-eQTLs, we split our overall sample set 1:1 into two sets by pedigrees creating separate discovery and replication sets, and identified cis- and trans- miR-eQTLs in each set. At discovery false discovery rates (FDRs) of <0.1, <0.05 and <0.01, the replication rates for cis -miR-eQTLs were 53%, 56% and 68% respectively, at a replication FDR<0.1, and 100% showed allele-specific directional effect concordance between the discovery and replication sets ( Fig. 1a,b ). In contrast, no trans -miR-eQTLs replicated (at FDR<0.1), although 91% of trans -miR-eQTLs showed allele-specific directional effect concordance in the discovery and replication sets ( Supplementary Fig. 4 ). Therefore, in the subsequent sections, we mainly report cis -miR-eQTLs identified in the overall FHS set (unadjusted for cell counts). 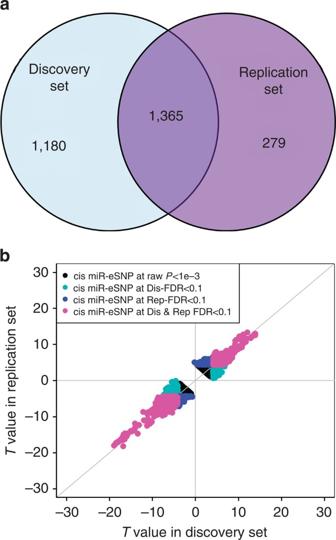Figure 1: Genome-wide identification ofcis-miR-eQTLs. (a) Venn diagram ofcis-miR-eQTLs identified in pedigree independent discovery (n=2,671) and replication sets (n=2,658). The number indicatedcis-miR-eQTLs identified in discovery, replication or both at FDR<0.1. (b)Tvalues ofcis-miR-eQTLs between discovery and replication groups. Figure 1: Genome-wide identification of cis -miR-eQTLs. ( a ) Venn diagram of cis -miR-eQTLs identified in pedigree independent discovery ( n =2,671) and replication sets ( n =2,658). The number indicated cis -miR-eQTLs identified in discovery, replication or both at FDR<0.1. ( b ) T values of cis -miR-eQTLs between discovery and replication groups. Full size image Genome-wide identification of miR-eQTLs At FDR<0.1 (corresponding P value threshold is 6.6 × 10 −5 ), we identified 5,269 cis- miR-eQTLs for 76 miRNAs (27% of interrogated expressed miRNAs) ( Fig. 2 ). These cis- miR-eQTLs were further pruned by removing redundant cis- miR-eQTLs with high linkage disequilibrium (LD). At a series of LD r 2 thresholds, that is, r 2 =0.2, 0.5, 0.7, 0.9 and 1, there were 283, 572, 982, 1,602 and 2,727 cis- miR-eQTLs retained. We further narrowed down the list to 52 peak cis -miR-eQTLs representing the single top cis -miR-eQTL for each miRNA or miRNA cluster shown in Supplementary Data 6 . Table 1 shows 16 of the 52 peak cis -miR-eQTLs with GWAS SNPs in the NHGRI GWAS Catalogue and the NHLBI GRASP data set [21] , [22] . A miRNA cluster is defined as a group of miRNAs located within 10 kb in the same chromosome (using the criteria described in www.mirbase.org ). miRNAs with higher heritability estimates were more likely to have cis -miR-eQTLs. All of the nine miRNAs with were found to have cis -miR-eQTLs. The top cis -miR-eQTLs tended to explain a greater proportion of the variance in the respective miRNA transcript as a function of increasing ( Fig. 3 ). When the heritability of miRNA transcripts increased from (0 to 0.1) to (0.3 to 1), the proportion of variance of the miRNA transcript explained by single cis -miR-eQTLs ( ) increased from 0.02 to 0.08 on average. 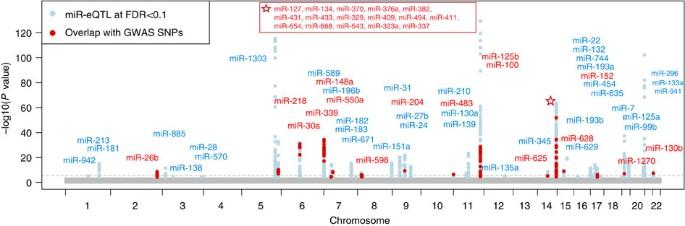Figure 2: Manhattan plot ofcis-miR-eQTLs. Genome-wide −log10 (P) value plots are shown for every interrogated miRNA (280 expressed miRNAs). Seventy six miRNAs havingcis-miR-eQTLs are labelled in this figure (for 52 unique peak loci). The horizontal dotted line indicates FDR<0.1 (corresponding toP<6.6 × 10−5).cis-miR-eQTL SNPs overlapping with GWAS SNPs reported in NHGRI GWAS Catalogue (http://www.genome.gov/gwastudies/)21and NHLBI GRASP database (http://apps.nhlbi.nih.gov/grasp/)22are shown in red. Figure 2: Manhattan plot of cis -miR-eQTLs. Genome-wide −log10 ( P ) value plots are shown for every interrogated miRNA (280 expressed miRNAs). Seventy six miRNAs having cis -miR-eQTLs are labelled in this figure (for 52 unique peak loci). The horizontal dotted line indicates FDR<0.1 (corresponding to P <6.6 × 10 −5 ). cis -miR-eQTL SNPs overlapping with GWAS SNPs reported in NHGRI GWAS Catalogue ( http://www.genome.gov/gwastudies/ ) [21] and NHLBI GRASP database ( http://apps.nhlbi.nih.gov/grasp/ ) [22] are shown in red. Full size image Table 1 Summary association results for 16 peak cis- miR-eQTLs having supporting GWAS evidence. 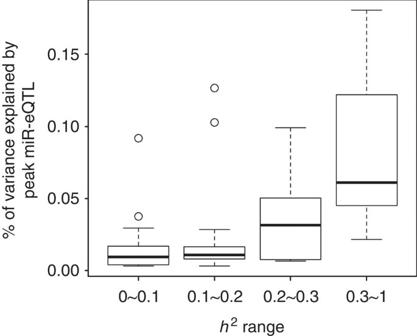Figure 3: The variance proportion of miRNA expression explained by singlecis-miR-eQTLs at different heritability levels. This figure was plotted by the boxplot function in the R library. The boxes indicate the interquartile range (IQR) of data between 75% (Q3) and 25% (Q1). The bars below and above each box indicate the data in Q1−1.5 × IQR and Q3+1.5 × IQR, respectively. Full size table Figure 3: The variance proportion of miRNA expression explained by single cis- miR-eQTLs at different heritability levels. This figure was plotted by the boxplot function in the R library. The boxes indicate the interquartile range (IQR) of data between 75% (Q3) and 25% (Q1). The bars below and above each box indicate the data in Q1−1.5 × IQR and Q3+1.5 × IQR, respectively. Full size image At FDR<0.10 (corresponding P value threshold is 1.0 × 10 −8 ), we identified 270 trans- miR-eQTLs for 15 miRNAs (5% of interrogated expressed miRNAs). Supplementary Figure 5 showed two-dimensional regional plot of cis- and tran- miR-eQTLs genome widely (unadjusted cell counts). 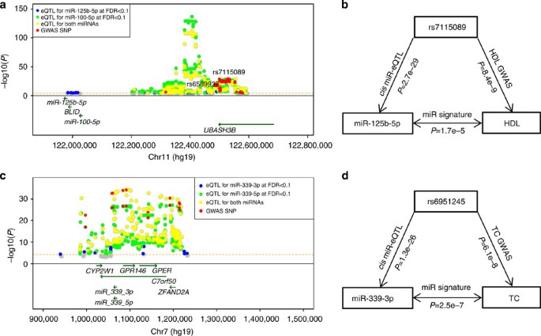Figure 5: Regional association plot ofcis-miR-eQTLs that were associated with GWAS SNPs. (a) miR-eQTLs for intergenic miRNAs miR-100-5p and miR-125b-5p, with GWAS SNPs for lipid traits, multiple sclerosis and rheumatoid arthritis. The highlighted SNP, rs7115089, is associated with both HDL and total cholesterol at GWASP<5 × 10−8by linear regression tests50; (b) the triangular relationships between SNP (that is, rs7115089), miRNA (that is, miR-125b-5p) and HDL cholesterol; (c) miR-eQTLs for intragenic miRNAs miR-339-3p and miR-339-5p, with GWAS SNPs for TC and LDL; (d) the triangular relationships between SNP (that is, rs6951245), miRNA (that is, miR-339-3p) and TC. –log10(P) indicates the –log10 transformed miRNA-SNP associationPvalues. Supplementary Data 7–8 showed trans- miR-eQTLs at FDR<0.1 identified in the overall samples of adjusted and unadjusted cell counts, respectively. We acknowledged those trans -miR-eQTLs that need to be validated in independent cohorts. cis -miR-eQTLs showing 5′ positional bias for miRNAs Among the 76 mature miRNAs with cis -miR-eQTLs, 49 (64%) were intragenic, located within annotated protein-coding genes (located in exons, introns or untranslated regions of the host genes) and 27 (36%) were intergenic. We discovered a marked positional bias of cis -miR-eQTLs, with many cis -miR-eQTLs located in the 5′-upstream region of the corresponding miRNA rather than within miRNA coding regions or the 3′-downstream regions. Among the 982 non-redundant (LD r 2 <0.7) cis- miR-eQTLs (representing 1,984 SNP-miRNA pairs), the relative distance of cis- miR-eQTLs to the corresponding mature miRNAs is shown in Fig. 4 and the relative distance of cis- miR-eQTLs to the transcriptional start site (TSS) is shown in Supplementary Fig. 6 . Specifically, for intragenic miRNAs, 418 cis- miR-eQTLs (493 SNP-miRNA pairs, 58%) were located in the 5′-upstream region of the corresponding primary miRNAs and 432 cis- miR-eQTLs (536 SNP-miRNA pairs, 63%) were in the region defined by 200 kb upstream to 100 kb downstream of the TSS. In contrast, for intergenic miRNAs, 238 cis- miR-eQTLs (825 SNP-miRNA pairs, 83%) were located in the 5′-upstream region of the corresponding primary miRNAs, and 125 cis- miR-eQTLs (487 SNP-miRNA pairs, 49%) were in the region defined by 500 to 300 kb upstream of the TSS ( Supplementary Data 9 ). 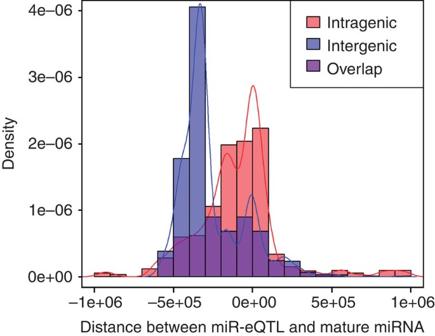There were 207 cis- miR-eQTLs (247 SNP-miRNA pairs, 29%) for intragenic miRNAs and 99 cis- miR-eQTLs (129 SNP-miRNA pairs, 13%) for intergenic miRNAs located within ±50 kb of the TSS of the corresponding miRNAs. Figure 4: The distribution of distance betweencis-miR-eQTLs and miRNA position. cis-miR-eQTLs for intergenic miRNAs are generally located further upstream than for intragenic miRNAs. The position of the first nuclear acid of the mature miRNA is marked as 0. The distribution statistics are based on 982 uniquecis-miR-eQTLs with LDr2<0.7. Figure 4: The distribution of distance between cis -miR-eQTLs and miRNA position. cis -miR-eQTLs for intergenic miRNAs are generally located further upstream than for intragenic miRNAs. The position of the first nuclear acid of the mature miRNA is marked as 0. The distribution statistics are based on 982 unique cis -miR-eQTLs with LD r 2 <0.7. Full size image Genomic features of cis -miR-eQTLs Most of the detected cis -miR-eQTLs are not located in protein-coding regions, that is, 39% of eQTLs in intronic and 57% in intergenic regions ( Supplementary Data 10 ). We found significant enrichment of cis -miR-eQTLs with expression regulatory elements ( Table 2 , Supplementary Data 11 and Supplementary Fig. 7 ), including CpG islands (2%), promoters (9%), enhancers (35%) and transcription factor (TF) binding regions (15%). We also found that cis -miR-eQTLs were enriched for miRNA mediated/targeted gene regulatory regions [23] , [24] . Table 2 Summary of human genome regulatory features of cis- miR-eQTLs. Full size table There were 1,066 (20%) cis- miR-eQTLs that overlapped with cis- mRNA-eQTLs identified in whole blood (enrichment P <1e−300 by hypergeometric test) [9] , [25] . An example is shown in Supplementary Fig. 8 ; 132 cis- miR-eQTLs (36%) for 12 intergenic mature miRNAs were also cis- mRNA-eQTLs for upstream protein-coding genes. We overlapped the 1 Mb region flanking the 132 cis- miR-eQTLs (chr14: 100.5–102.5 Mb) with the regulatory feature tracks downloaded from UCSC Genome Browser (genome.ucsc.edu). Supplementary Figure 8 showed that the nearby regions of the 132 cis- miR-eQTLs for those 12 miRNAs overlap with Enhancer active region (chr14:101,100 kb–101,200 kb, H3K4Me1 and H2K27AC track, marked in lightyellow rectangle). The highly unmethylated status of GM12878, K562, HeLa-S3 and HepG2 cell lines are in chr14:101,400 kb–101,600 kb upstream of those cis- mRNA-eQTL miRNAs (CpG Methylation by Methy450K Bead Arrays from ENCODE/HAIB track, marked by pink colour). We also discovered 11 intragenic mature miRNAs share cis- eQTLs with their host mRNA genes ( Supplementary Data 12 ). For cis- miR-eQTLs that overlapped with cis- mRNA-eQTLs, we performed conditional analysis to test if the associations between SNPs and miRNAs remained significant when conditioning on the corresponding mRNA expression levels using results from 5024 FHS participants with genotype, and miRNA, and mRNA expression data. As show in Supplementary Data 13 , we found 923 cis- miR-eQTLs for 3,384 miRNA-SNP association pairs (87%) that remained significant at FDR<0.1 (corresponding P <6.6 × 10 −5 ) when conditioning on mRNA expression levels. These findings indicate that cis genetic variants may affect expression levels of neighbouring miRNAs and mRNAs. cis -miR-eQTLs and miRNA signatures for complex traits We linked the cis -miR-eQTLs with GWAS SNPs in the NHGRI GWAS Catalogue and the NHLBI GRASP data set [21] , [22] . Among 5,269 cis -miR-eQTLs, 243 cis -miR-eQTLs (for 31 miRNAs) overlapped with GWAS SNPs, including SNPs associated with multiple complex traits ( Table 1 , Fig. 2 , and regional association plots for several traits including height, menarche, platelet count and lipid levels are shown in Supplementary Fig. 9 ). For miRNAs with cis -miR-eQTLs showing association with complex traits in GWAS, we further tested if expression of these miRNAs in FHS participants was associated with the corresponding traits. We discovered a number of miRNAs that showed differential expression in relation to the complex traits that correspond to the traits associated with their eQTLs in GWAS ( Table 1 ). For example ( Fig. 5a,b ), among cis -miR-eQTLs of miR-100-5p and miR-125b-5p, we found 28 cis -miR-eQTLs (that is, GWAS SNPs) that were associated in GWAS with lipid traits (high-density lipoprotein (HDL) cholesterol, low-density lipoprotein (LDL) cholesterol, total cholesterol (TC) and triglycerides (TGs)), 1 (rs7941030) with multiple sclerosis and 1 (rs1216554) with rheumatoid arthritis. These eQTLs are located ~519 kb upstream of their two associated miRNAs. We also found that miR-125b-5p showed differential expression in relation to plasma TC ( P =0.005, by linear regression tests, see Methods) and HDL cholesterol ( P =1.68e−5) and miR-100-5p showed differential expression in relation to HDL cholesterol ( P =0.039). Another example ( Fig. 5c,d ) is for miR-339-3p and miR-339-5p, which are located in an intron of c7orf50 . Among the 282 cis -miR-eQTLs SNPs of miR-339-3p and 279 cis -miR-eQTLs of miR-339-5p, 8 were associated with TC and 3 with LDL cholesterol. We also found that expression of miR-339-3p was associated with TC ( P =2.5e−7). These results establish links between SNPs affecting both miRNA expression levels and complex traits. Mendelian randomization (MR) tests provided evidence that four cis -miR-eQTLs SNPs (rs6951245, rs11763020, rs1997243 and rs2363286) alter the expression levels of miR-339-3p and miR-339-5p, and in turn affect interindividual variability of TC levels (causal P <0.05). Figure 5: Regional association plot of cis -miR-eQTLs that were associated with GWAS SNPs. ( a ) miR-eQTLs for intergenic miRNAs miR-100-5p and miR-125b-5p, with GWAS SNPs for lipid traits, multiple sclerosis and rheumatoid arthritis. The highlighted SNP, rs7115089, is associated with both HDL and total cholesterol at GWAS P <5 × 10 −8 by linear regression tests [50] ; ( b ) the triangular relationships between SNP (that is, rs7115089), miRNA (that is, miR-125b-5p) and HDL cholesterol; ( c ) miR-eQTLs for intragenic miRNAs miR-339-3p and miR-339-5p, with GWAS SNPs for TC and LDL; ( d ) the triangular relationships between SNP (that is, rs6951245), miRNA (that is, miR-339-3p) and TC. –log10( P ) indicates the –log10 transformed miRNA-SNP association P values. Full size image On the basis of extensive integrated analyses of miRNA expression and genetic variants genome wide in 5,239 individuals, we established a clear pattern of heritability of blood miRNA expression, and identified a substantial number of miRNAs that are controlled by cis genetic regulatory elements. Our results for cis -miR-eQTLs were highly replicable; in contrast, trans -miR-eQTLs were not replicable. Previously reported miR-eQTLs were identified in studies with small sample sizes ( n <200) and revealed a few miR-eQTLs. For example, Borel et al. [14] using umbilical cord blood from 180 newborns, identified only 12 cis -miR-eQTLs at FDR<0.5. In another study, no cis -miR-eQTLs were found in 176 lymphoblastoid cell lines from European and African ancestry samples [15] . Proxy SNPs of two cis -miR-eQTLs that we identified (rs2187519 for miR-100 and rs7797405 for miR-550) were reported by Borel et al. [14] (rs10750218 as a proxy for rs2187519 and rs12670233 for rs7797405 are in modest LD at r 2 =0.29 and r 2 =0.48, respectively). As our data are from a well-powered multi-generation study, we were able to assess narrow sense heritability ( ) of each miRNA expression trait. By comparing the overall heritability of the miRNAs and single cis -miR-eQTLs, we discovered that miRNAs with higher heritability were more likely to have cis -miR-eQTLs. When the heritability of miRNA transcripts increased, the proportion of variance of the miRNA transcript explained by single cis -miR-eQTLs ( ) increased as well. Our heritability study of mRNA expression traits revealed single cis -mRNA-eQTLs that explained 33–53% of variances in corresponding mRNA expression levels [26] . In contrast, single cis -miR-eQTLs explained much less proportion of variances in corresponding miRNA expression levels (~1.3% on average). In contrast to the functional annotation of cis- mRNA-eQTLs, most of which are within ~250 kb of mRNA TSS and without 5′ or 3′ positional bias [13] , we discovered that most cis -miR-eQTLs (58% for intragenic miRNAs and 83% for intergenic miRNAs) are located upstream of mature/primary miRNAs. For intergenic miRNAs, a significant fraction of cis -miR-eQTLs are quite far upstream (~300–500 kb). Distal regulatory elements can interact with the proximal elements that regulate miRNA expression [27] . In our results, we found that a significant fraction of cis -miR-eQTLs are distal, suggesting that variants in far upstream regions may play important roles in miRNA transcription. In addition, our results revealed that distal cis -miR-eQTLs explained a modest proportion (~1.3% on average) of variance in miRNA expression levels. We speculate that the mild effects of cis -miR-eQTLs on miRNA expression result from evolutionary selection to stabilize the biological functions mediated by miRNAs. Genetic variants that modify chromatin accessibility and transcription factor binding are a major mechanism through which genetic variation leads to expression differences for protein-coding genes in humans [28] . The investigation of regulatory mechanisms of miRNA transcription is still evolving. Genomic feature analyses of cis -miR-eQTLs reveal that a large proportion of cis -miR-eQTLs are located in regulatory elements such as CpG islands (2%), promoters (9%), enhancers (35%) and TF binding regions (15%). We also discovered that cis -miR-eQTLs show a significant enrichment for mRNA-eQTLs and 87% of cis -miR-eQTLs that are also mRNA-eQTLs remained significant when conditioning on the corresponding mRNA expression levels. For example, as shown in Supplementary Fig. 8 , 132 cis -miR-eQTLs (36%) for 12 intergenic miRNAs were also cis -mRNA-eQTLs for upstream protein-coding genes. This finding suggests that genetic variants may influence the expression of both miRNAs and nearby protein-coding genes. These eQTL regulatory effects may act via modified chromatin accessibility, transcription factor binding affinity or DNA methylation. The mechanisms of transcriptional regulation of intragenic miRNAs are more complex than intergenic miRNAs, as intragenic miRNAs may mirror the regulatory mechanisms of their host genes, or be transcribed independently as a consequence of their unique promoter regions [29] . We identified 11 mature miRNAs from intragenic miRNAs that share cis eQTLs with their host protein coding genes ( Supplementary Data 12 ). Among the cis -mRNA-eQTL miRNAs, 15 miRNAs have alternative intronic promoters (alternative intronic promoters were from ref. 29 ). We overlapped the cis -miR-eQTLs and expression regulatory elements annotations from ENCODE nearby regions of each miRNA (±50 kb). We found, in some examples ( Supplementary Fig. 10 ), cis -miR-eQTLs near alternative intronic promoter regions demonstrated promoter and enhancer activities and were highly un-methylated in some cell lines. Our findings provide a guide for further functional studies of transcriptional elements of miRNAs. We identified numerous cis -miR-eQTLs that are associated with complex diseases/traits in GWAS ( Table 1 ). Equally noteworthy, we found several examples in which the miRNAs associated in cis with these GWAS SNPs were associated with the corresponding trait (for example, three-way association of HDL cholesterol with its GWAS SNP, rs7115089 and with the corresponding miR-125b-5p). A single miRNA may target hundreds of protein-coding genes. Therefore, the effect of genetic variants on miRNAs can play an important regulatory role in mediating the targeted protein-coding genes, as well as complex phenotypes. We speculate that some of the protein-coding genes targeted by miRNAs may also be involved in the cellular pathways related to the trait. For example, miR-125b-5p expression was associated with HDL cholesterol ( P =1.7 × 10 −5 , by a linear regression test). In a parallel project focusing on differentially expressed mRNAs in association with lipid levels, we found 17 genes targeted by miR-125b-5p (9% of miR-125b-5p targeted genes in miRTarBase [24] ) that showed differential expression in association with HDL cholesterol (at P <0.05 corrected for ~18,000 genes, by a linear regression test) [30] . Some of these genes are involved in metabolic processes, for example, PRDX2 , which was downregulated in association with HDL cholesterol ( P =1.1 × 10 −15 , by a linear regression test). Further studies and biological experiments are needed to investigate whether these cis- miR-eSNPs affect the corresponding miRNA targeting genes. In summary, our genome-wide miR-eQTL mapping study provides new insights into the genetic regulation of miRNA transcription and the roles of miRNAs in complex diseases. Our findings may help to identify new opportunities for drug treatment or diagnosis of human diseases. Study populations The FHS is a community-based study that began enroling participants in 1948. In 1971, the offspring and offspring spouses (the offspring cohort) of original FHS cohort participants were recruited and they have been examined every 4 to 8 years [31] . From 2002 to 2005, the adult children of the offspring cohort participants (the third generation cohort) were recruited and examined [32] . In this study, we investigated 2,272 offspring cohort attendees at examination cycle 8 (2005–2008) and 3,057 third generation cohort attendees at examination cycle 2 (2008–2010). This study was approved under the Boston University Medical Center protocol H-27984. Written informed consent was obtained from each participant. miRNA expression profiling miRNAs were measured from venous blood samples obtained from participants after overnight fasting. Whole blood samples (2.5 ml) were collected in PAXgene Blood RNA tubes (Qiagen, Valencia, CA, USA) and frozen at −800 °C. Total RNA was isolated from the frozen PAXgene Blood RNA tubes (Asuragen, Inc. Austin, TX, USA) and a 2100 Bioanalyzer Instrument (Agilent, Santa Clara, CA, USA) was used for RNA quality assessment. Isolated RNA samples were converted to complementary DNA using TaqMan miRNA Reverse Transcription Kit and MegaPlex Human RT Primer Pool Av2.1 and Pool Bv3.0. (Life Technologies, Foster City, CA, USA) in a 384-well Thermal Cycler. The complementary DNA samples were PreAmplified using TaqMan PreAmp Master Mix and PreAmp Primers, Human Pool A v2.1 and Pool B v3.0 (Life Technologies). Quantitative reverse transcription PCR (qRT–PCR) reactions were performed with the BioMark System using (Fluidigm, South San Francisco, CA, USA) TaqMan miRNA Assays (Life Technologies). As described in the published literature, measurement of RNA by qRT–PCR is reliable and has high specificity and sensitivity [33] , [34] , [35] , [36] . The initial miRNA list encompassed all commercially available TaqMan miRNA assays obtainable at the start of the project (754 mature miRNAs). These miRNAs were initially assayed for measurement feasibility in RNA samples from 450 FHS participants. All qRT–PCR reactions were performed in the BioMark Real-Time PCR system using the following protocol: 10 min at 95 °C, 15 s at 95 °C and 1 min at 60 °C for 30 cycles. Single copy can be detected with BioMark system at 26–27 cycle thresholds. For replicates >95% of the data points had coefficients of variation <10% (mean ~4%). miRNA normalization We normalized miRNA expression using a model that adjusts raw miRNA cycle threshold (Ct) values for 4 technical variables: isolation batch (50 batches), RNA concentration, RNA quality (defined as RNA integrity number) and RNA 260/280 ratio (ratio of absorbance at 260 and 280 nm; measured using a spectrophotometer). Histograms ( Supplementary Fig. 11 ) show that this model explains 20–60% of variability of raw miRNA measurements for 80% of miRNAs Genotyping DNA was isolated from buffy coat or from immortalized lymphoblast cell lines. Genotyping was conducted with the Affymetrix 500 K mapping array and the Affymetrix 50 K gene-focused MIP array, using previously described quality control procedures [37] . Genotypes were imputed to the 1000 Genomes Project panel 19 of ~36.3 million variants using MACH [38] . We filtered out SNPs with MAF<0.01 and imputation quality ratio <0.1 (the imputation quality ratio is denoted by the ratio of the variances of the observed and the estimated allele counts), resulting in 9.8 × 10 6 SNPs (~10 million SNPs) that were eligible for further miR-eQTL testing. miR-eQTL mapping Because of the computational burden of running linear mixed effects (LMEs) models for ~10 million (SNPs) × 280 miRNAs (miRNAs expressed in >200 samples), we adapted a two-step analysis strategy. Step 1: linear regression was used to model the association between miRNA Ct values ( ) and the imputed SNP genotypes—adjusted for age, sex, cohort and technical covariates—yielding results for roughly 280 miRNAs × 10 million SNPs, as shown in Equation (1). Associated SNP–miRNA pairs residing within 1 Mb of the mature miRNA ( cis ) and those residing more than 1 Mb away ( trans ) were identified separately. We chose liberal P value thresholds to pre-filter the miR-eQTLs, at P <1 × 10 −3 for cis and P <1 × 10 −5 for trans . These P value thresholds were chosen to ensure that miR-eQTLs at a FDR <0.1 were not omitted as a result of this pre-filtering step. Step 2: we used a linear mixed model [39] to recalculate the associations of SNPs and miRNA expression levels for the pre-selected eQTLs from step 1, adjusted for age, sex and technical covariates as fixed effects and a familial correlation matrix (FAM) as the random effect using the lmekin() function of Kinship Package ( http://cran.r-project.org/web/packages/kinship/ ) [39] , as shown in Equation (2). In Equations (1) and (2), ε is the error term for each independent observation. Genome coordinate annotation for miRNAs used miRbase v20 (mirbase.org), and for SNPs we used the February 2009 assembly of the human genome (hg19, GRCh37 Genome Reference Consortium Human [37] ). Based on the coordinates of 280 mature miRNAs and 9.8 × 10 6 SNPs, we estimated there were 13,935,272 (1.4 × 10 7 ) potential SNP-miRNA pairs, where the SNP was located within 1 Mb on either side of the corresponding mature miRNA. We estimated there were 1.4 × 10 7 potential cis SNP–miRNA pairs, and 2.7 × 10 9 (that is, 280 × 9.8 × 10 6 −1.4 × 10 7 ) potential trans SNP–miRNA pairs. We used the Benjamini–Hochberg method [40] to calculate FDR for cis- and trans- miR-eQTLs by correcting for 1.4 × 10 7 potential cis SNP–miRNA pairs and 2.7 × 10 9 potential trans SNP–miRNA pairs, respectively. We selected an FDR threshold of 0.1, corresponding to P <6.6 × 10 −5 for cis- and P <1.0 × 10 −8 for trans- miR-eQTLs. For identified cis- miR-eQTLs at FDR<0.1, we used Fragmented Exhaustive Search for TAgSNPs (FESTA) [41] to select non-redundant miR-eQTLs based on a series of LD r 2 thresholds 0.2, 0.5, 0.7 0.9 and 1. FESTA used a mixture of search techniques to partition the whole SNP set into disjointed precincts and selected a tag SNP for each SNP block, which represented a set of SNPs at a LD r 2 >threshold [41] . To estimate the replicability of miR-eQTLs, we split the overall sample set at a 1:1 ratio into discovery and replication sets. The discovery and replication sets represent independent pedigrees to ensure that individuals in the two sets were unrelated. We used the methods described above to identify miR-eQTLs in the discovery and replication sets separately. We evaluated the concordance of effect sizes of cis - and trans -miR-eQTLs in the discovery and replication sets. We identified eQTLs at FDR<0.1 in the discovery set, and attempted to replicate them in the replication set. mRNA expression data Whole blood samples (2.5 ml) were collected in PAXgene tubes by Asuragen, Inc. (PreAnalytiX, Hombrechtikon, Switzerland). Total RNA was isolated according to the company’s standard operating procedures for automated isolation of RNA from 96 samples in a single batch on a KingFisher 96 robot. Then 50 ng RNA samples were amplified using the WT-Ovation Pico RNA Amplification System (NuGEN, San Carlos, CA, USA) as recommended by the manufacturer in an automated manner using the genechip array station. RNA expression was conducted using the Affymetrix Human Exon Array ST 1.0 (Affymetrix, Inc., Santa Clara, CA, USA). The core probe sets were annotated using the Affymetrix annotation files from Netaffx ( www.netaffx.com,HuEx-1_0-st-v2.na29.hg18.probeset.csv ). The raw gene expression data were at first preprocessed by quartile normalization. Then the robust multi-array average values of every gene (17,318 measured genes) were adjusted for a set of technical covariates, for example, chip batch by fitting LME models. Imputed blood cell counts (that is white blood cell (WBC), red blood cell (RBC), platelet, lymphocyte, monocyte, eosinophil, and basophil) (Joehanes R, in preparation) were also evaluated as covariates and adjusted if deemed significant, as detailed below. The residuals were retained for further analysis. Matching cis- miR-eQTLs with cis- mRNA-eQTLs We overlapped the cis- miR-eQTLs at FDR<0.1 reported in this study with cis- mRNA-eQTLs at FDR<0.1 identifed by refs 9 , 25 . Hypergeometric test was used to evaluate if cis- miR-eQTLs were significantly enriched for cis- mRNA-eQTLs. For those overlap eQTLs, that is, cis- miR-eQTLs that were also cis- mRNA-eQTLs, we used the same linear mixed regression model as described in ‘miR-eQTL mapping’ section to re-analyze the associations between genotypes and miRNA expression levels but conditional regression on corresponding mRNA expression levels. Estimating effects of cell counts in the miR-eQTLs Since the miR-eQTLs in whole blood may be driven by cellular composition, we compared the miR-eQTLs in 2,138 individuals with measured cell counts before and after correction for cell count effects ( Supplementary Fig. 3 ). Differential cell counts and proportions in whole blood were measured in 2,138 individuals in the FHS third generation cohort, including seven cell types, WBC, RBC, platelet, neutrophil, lymphocyte, monocyte, eosinophil and basophil. The cell counts and proportions for 5,024 FHS participants were estimated using mRNA expression values by partial least squares regression prediction. The estimated cell count proportion values are highly consistent with the measured cell counts proportion values (Joehanes R, unpublished data, 2014). We did not find any evidence that cell counts affected the miR-eQTLs; however, we cannot exclude small effects from cell counts. Therefore, we report miR-eQTLs unadjusted for cell counts in our main results, and secondarily report miR-eQTLs adjusted for imputed cell counts (that is, WBC, RBC, platelets, lymphocytes, monocytes, eosinophils and basophils) in Supplementary Data 5 . Please note that there were 215 samples without mRNA expression data; therefore, the maximum sample size of analyses unadjusted for cell counts is 5,239 and the maximum sample size of analyses adjusted for cell counts is 5,024. Estimating the heritability of miRNA expression levels To estimate the narrow-sense heritability of the expression for a specific miRNA (denoted as ), we used the model as shown in Equation (3). Here age, sex and technical covariates were included as fixed effects, FAM was the familial correlation matrix included as the random effect. FAM-represented additive polygenic genetic effects [39] . ε is the error term for each independent observation. was the proportion of the additive polygenic genetic variance ( ) among the total phenotypic variance of miRNA expression: . We estimated for every miRNA expression trait (247 miRNAs expressed in >1,000 samples) using the lmekin() function of Kinship package ( http://cran.r-project.org/web/packages/kinship/ ) [39] . Estimating proportion of variance in miRNAs attributable to miR-eQTLs To estimate the proportion of variance in a single miRNA trait that is attributable to a single miR-eQTL (denoted as ), we used the following two models: Full model: Null model: Here age, sex, cohort (offspring cohort and the third generation cohort in the FHS) and technical covariates were included as fixed effects, FAM was the familial correlation matrix included as the random effect. ε is the error term for each independent observation. The proportion of variance in a single miRNA trait that is attributable to a single miR-eQTL was denoted as and was calculated as follows: where was the total phenotypic variance of a miRNA expression trait; and were the polygenic and error variances, respectively, when modelling with the tested miR-eQTL; and were the polygenic and error variances, respectively, when modelling without the tested miR-eQTL. The lmekin() function in the Kinship package [39] was used to estimate . Identification of differentially expressed miRNAs for complex traits We used the NHGRI GWAS Catalogue ( http://www.genome.gov/gwastudies/ ) [21] and NHLBI GRASP database ( http://apps.nhlbi.nih.gov/grasp/ ) [22] to annotate complex trait associated miR-eQTLs. The cis -miR-eQTLs identified in this study were compared with SNPs in the NHGRI GWAS Catalogue and NHLBI GRASP GWAS results for SNPs at P <1 × 10 −5 . For the complex traits that could be mapped with cis -miR-eQTLs (and also were measured in the FHS), including menarche, lipids (HDL cholesterol, TG and TC), type II diabetes mellitus (T2D) and glucose level, we used linear mixed models to test their association with miR-eQTL miRNAs in FHS individuals. These phenotypes were ascertained at examinations 8 and 2 for the offspring and the third generation cohorts, respectively. We identified differentially expressed miRNAs associated with HDL cholesterol, TC, TG, T2D and glucose after accounting for age, sex, cell counts and technical covariates (see ‘miRNA normalization’ in methods) and family structure in LME models implemented in the lmekin function [39] . Differentially expressed miRNA associated with age at menarche were tested in LME models (lmekin) after accounting for birth year, cell counts, technical covariates and family structure. miRNA TSS and promoter regions The transcriptional regulatory mechanisms affecting miRNA expression are unclear. There are technical barriers to the precise identification of primary miRNAs, TSSs and promoter regions for most mature miRNAs [29] . Recently, Marsico et al. [29] and Chen et al. [42] predicted miRNAs TSSs. Their results were incorporated with the results from previous similar studies [43] . However, by comparing the TSS positions identified by these two studies, there was, on average, 55 kb distance difference between TSSs positions to the corresponding mature miRNAs. Therefore, in our analysis, we annotated the miRNA TSSs collected and predicted by these two studies. The predicted promoter annotations for miRNAs were obtained from Marsico et al. [29] which were screened within ±50 kb from the TSSs for each miRNA. Functional annotation of cis -miR-eQTLs We annotated the genomic features cis -miR-eQTLs ( n =5,269) using HaploReg [44] , which integrates results from ENCODE [20] . The overlap of cis -miR-eQTLs with ENCODE annotated SNPs in promoter, enhancer and TF binding sites were retrieved ( Supplementary Data 11 ). For enrichment tests of functional SNPs in cis -miR-eQTLs identified in this study, we downloaded regulatory tracks contained in the UCSC Genome Browser, including ENCODE histone modification sites, and TF and CTCF binding sites in lymphoblastoid cell lines (GM12878), Open Regulatory Annotation (ORegAnno) [45] , UCSC CpG islands and long intergenic non-coding RNA [46] . We also downloaded other regulatory tracks, including experimentally validated miRNA targets from TARbase [47] , and experimentally supported miRNA-mediated gene regulatory sites from Patrocles [23] . Binominal tests were used to evaluate if the identified cis -miR-eQTLs set (5,269 cis -miR-eQTLs) showed enrichment for regulatory SNPs for each track (methods described by ref. 13 ). We further determined whether or not the detected cis -miR-eQTLs SNPs were enriched for promoter, enhancer or protein binding regions on the genome. To do so, we annotated all cis -miR-eQTLs ( n =5,269) using HaploReg [44] , which integrates results from ENCODE [20] . We examined enrichment in nine different cell lines (that is, GM12878, H1-hESC, HepG2, HMEC, HSMM, HUVEC, K562, NHEK and NHLF). The null distributions of eQTLs were generated using a permutation strategy by randomly selecting equal number of SNPs ( n =5,269) 100 times. The pools of candidate SNPs for the permutation were from 1000-genomes imputed SNPs with MAF >0.01 and imputation quality ratio >0.1. To match the distribution of MAFs of the permutation SNPs (the permutation-SNPs set) with the cis -miR-eQTLs SNPs (the tested-SNPs set), we categorized MAF into four categories: MAF of (0.01, 0.05), (0.05, 0.1), (0.1, 0.2) and (0.2, 0.5). For each MAF category, we kept the proportion of SNPs in the permutation-SNPs set equal to the proportion of SNPs in the tested-SNPs set. In the four MAF categories, the proportions of SNPs are 3%, 7%, 19% and 71% respectively. The average of the overlap between permutation and regulatory region SNPs (that is SNPs in promoter, enhancer and protein binding regions) was compared with the overlap between the tested SNPs and regulatory region SNPs. MR test We used a two-stage least squares (2SLS) MR method [48] to estimate the causal relationships between miRNAs and complex traits measured in FHS participants; the traits analyzed included menarche, lipids (HDL, TG and TC), T2D and glucose, using cis- miR-eQTLs as instrumental variables. MR was only performed in the pre-filtered SNP-miRNA-trait pairs, when a SNP was a cis- miR-eQTL and also present in NHGRI GWAS Catalogue ( http://www.genome.gov/gwastudies/ ) [21] or in the NHLBI GRASP database ( http://apps.nhlbi.nih.gov/grasp/ ) [22] , and the miRNA showed differential expression in relation to the corresponding trait at P <0.05 in FHS participants. To determine the strength of the genetic instrument, an F-statistic in a linear regression model was derived from the proportion of variation in the miRNA expression levels (miRNA Ct values) that was explained by the corresponding cis- miR-eQTL, by modelling age, sex, family structure and four technical variables as covariates (see in the miRNA normalization section). cis- miR-eQTLs with an F-statistic <10, indicating a weak instrument, were excluded. The first stage of the 2SLS method involves using a linear regression of the modifiable exposure (miRNA) on the instrumental variable (SNP) and covariates, and saving the predicted miRNA values. In the second stage, the outcome (complex trait) is regressed on the predicted miRNA values. The regression coefficient obtained in the second stage can be interpreted as being the causal effect of the exposure (miRNA) on the outcome (complex trait). The Durbin–Wu–Hausman test [49] is used to estimate whether the estimates derived from the first and second stage of the 2SLS are consistent. Accession codes: The mRNA and microRNA expression data of patient samples have been deposited in dbGaP ( http://www.ncbi.nlm.nih.gov/gap ) under the accession number phs000007. How to cite this article: Huan, T. et al. Genome-wide identification of microRNA expression quantitative trait loci. Nat. Commun. 6:6601 doi: 10.1038/ncomms7601 (2015).